Fundamental limitations for quantum and nanoscale thermodynamics The relationship between thermodynamics and statistical physics is valid in the thermodynamic limit—when the number of particles becomes very large. Here we study thermodynamics in the opposite regime—at both the nanoscale and when quantum effects become important. Applying results from quantum information theory, we construct a theory of thermodynamics in these limits. We derive general criteria for thermodynamical state transitions, and, as special cases, find two free energies: one that quantifies the deterministically extractable work from a small system in contact with a heat bath, and the other that quantifies the reverse process. We find that there are fundamental limitations on work extraction from non-equilibrium states, owing to finite size effects and quantum coherences. This implies that thermodynamical transitions are generically irreversible at this scale. As one application of these methods, we analyse the efficiency of small heat engines and find that they are irreversible during the adiabatic stages of the cycle. One of the most basic quantities in thermodynamics is the Helmholtz free energy with T the temperature of the ambient heat bath that surrounds the system, S ( ρ ) the entropy of the system and its average energy. It tells us whether a system at constant volume and in contact with a heat bath can make a spontaneous thermodynamical transition from one state to another. A transition can only happen if the free energy of the final state is lower than that of the initial state. The difference in free energy between the initial and final state is also the amount of work that can be extracted from a system in a thermal bath. It also gives the amount of work required to perform the reverse process, as thermodynamics at the macroscopic scale is reversible. However, the free energy is only valid in the thermodynamical limit—when ρ is composed of many particles and is classical, in the sense that it is in a state that is a probabilistic mixture of different energies. However, thermodynamical effects are not only important in the macroscopic regime—they are becoming increasingly important as we probe and manipulate small systems from the micro up to the mesoscopic scale. Already, molecular motors and micro-machines [1] , [2] , [3] , [4] , [5] , [6] , [7] , [8] , [9] have been constructed in the lab [1] , [10] , [11] , [12] and thermodynamical effects are increasingly important in quantum devices and in the construction of quantum computers and memory [13] , [14] , [15] . Likewise, quantum effects have implications for thermodynamics [16] , [17] , [18] . In this article, we derive necessary and sufficient conditions for thermodynamical state-to-state transitions, which are valid even when the thermodynamical limit is not taken, and even when the system is quantum. We call these conditions thermo-majorization. As a special case of this more general result, we derive two free energies valid in this regime. We also quantify the extent to which general state transformations are irrversible, and derive a criteria for when transitions between two states block-diagonal in energy eigenbasis can be made reversible in the micro-regime. We find that there are particular processes that approach the ideal efficiency, provided that certain special conditions are met. Our most basic result concerns the state of a micro-system, which is out of equilibrium, and we ask first how to define microscopic work, and then we provide the optimal amount of work that can be drawn from the system when in contact with a heat bath, as well as the amount of work required for the reverse process (the work of formation). The obtained amount of work is given by a version of the relative entropy distance of the state from the Gibbs state. Similarly, the work needed to create a system is given by another version of the relative entropy distance to the Gibbs state. These two cases are examples of our full thermo-majorization result, which includes characterization of all possible transitions between states block-diagonal in the energy eigenbasis in the presence of a heat bath. Conceptual prerequisites In the macroscopic regime, the standard free energy can be expressed by means of the relative entropy [19] , and this can be used to compute the work drawn from non-equilibrium states [20] , [21] . However, it is surprising that in the micro-regime, where fluctuations may dominate, the distillable work and work of formation can also be expressed as relative entropies, albeit very different ones. This is because in the micro-regime, one has a single system with large fluctuations, and it is not at all clear that one can draw work deterministically, as one does in the macroscopic case. One might have imagined that one need to look at the non-deterministic case where one sometimes succeeds in drawing work, and sometimes does not. This approach, while certainly of interest, has the disadvantage that without deterministic work extraction, it can be difficult to separate work from the entropy stored with the work, as if one is not almost certain to draw work, the work will be inherently noisy. To make the distinction between work and noise, one then invariably looks at running a thermodynamic cycle many times, and this does not allow one to fully consider individual systems. In contrast, here, we are able to make strong statements about what will happen to a single system. Our results were possible owing to combining a number of existing concepts. The case of manipulation of entropy, and deterministic transitions when the Hamiltonian is trivial, was undertaken in Horodecki et al . [22] , where transition criteria and work extraction were given by majorization conditions. This can be considered a resource theory of ‘purity’ or entropy. In Dahlsten et al . [23] , a probability of failure was allowed for extracting work, allowing work to be quantified by smooth entropies, and this was extended in Del Rio et al . [18] to the case where one only wants to extract work from one subsystem of a bipartite state, while preserving the other subsystem. In these three cases, as energy was essentially decoupled from entropy, work extraction was a purely information-theoretic task—defined as going from a mixed state to a pure state—enabling a generalization of Landauer’s principle, saying that a pure state of a two-level system without a Hamiltonian is equivalent to kT ln 2 of work. Indeed, one links the concept of work to entropy change, simply through Landauer’s principle. However, thermodynamics is not merely the study of entropy, but rather the interplay between energy and entropy. Entropy is only half the picture. A key tool we will need to use is a resource theory that combines the resource theory of purity with that of ‘asymmetry’, which is the study of manipulations constrained by superselection rules [24] , of which energy conservation is a special case. Combining these two resource theories allows one to study thermodynamics in all its generality. A paradigm was presented in Janzing et al . [25] and we shall employ its components as a resource theory here, but with two new twists—first, while keeping the system microscopic, we consider its interaction with a large heat bath. This allows us to combine the above-mentioned approaches together with the quantum information theory of resources, to obtain a novel theory of thermodynamics in the micro-regime. Second, we will add a work system into the picture, which will allow us to define work as the process of raising an energy level of this work system. The skeleton of our construction is the theory of resources, and in a parallel paper [21] , we show how it reconstructs thermodynamics in the macroregime in the particular case of many identical copies of a micro-system. The present paper concerns itself with the micro-regime. Remarkably, even when we have a non-trivial Hamiltonian acting on our system, and manipulate systems through a non-trivial interaction Hamiltonian between the system and reservoir, we still find that work extraction and formation are given by elegant information-theoretic quantities. Thermal Operations We will first consider a quantum system with a fixed Hamiltonian H and eigenstates of energy E given by | E , g ›, in contact with a heat bath. We are interested in the types of state transitions that are allowed and, in particular, our ability to use the system as a resource to extract work. We will then consider the case where the Hamiltonian of the initial and final state is not the same, so that the system undergoes a non-cyclic evolution. Instead of considering macroscopic work (the pushing out of a piston or the raising of a weight), we consider microscopic work—for example, the exciting of an atom from its ground state to an excited state ( Fig. 1 ). We can thus use a two-level system to store work. As the amount of extractable work can be small, we require precise accounting of all sources of energy. We thus consider a paradigm where extraction of work, and other operations, must be done using energy-conserving operations [21] , [25] , so that any energy that is transferred to or from the resource system and heat bath is transferred from or to the system that stores work. We do not impose any additional constraints, as we wish to explore fundamental limitations on what can be accomplished on work extraction and formation. We call the class of operations that are allowed Thermal Operations—a fuller discussion of which is contained in Supplementary Note 1 , including how it is related to other natural paradigms. This casts thermodynamics as a resource theory [21] , [22] , [25] , [26] , [27] , [28] , which allows us to exploit some mathematical machinery from information theory. Thermodynamics is then viewed as a theory involving state transformations in the presence of a thermal bath. The extraction or expenditure of work can be included in such a paradigm, because it is equivalent to a state transformation—the state of the work qubit is raised or lowered from one energy eigenstate to another. 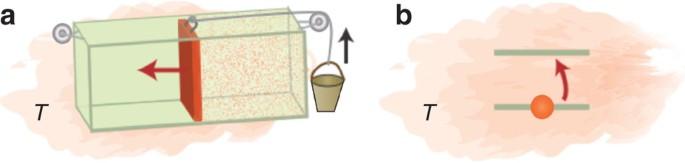Figure 1: Macroscopic and microscopic work. (a) A macroscopic heat engine that performs work by lifting a heavy weight a certain height. (b) In the quantum or micro-regime, we can think of work as the ability to excite a two-level system from one energy state to a higher one. Having many of these atoms would allow us to perform macroscopic work—for example, we could use the atoms in a laser. An amount of workWcan be used to produce a transition from the state |00| to the state |11|, with Hamiltonian(we call such a two-level system the work qubit or wit). We can use such a system as a basic work storage unit, as our results will not depend on what physical system is used. Figure 1: Macroscopic and microscopic work. ( a ) A macroscopic heat engine that performs work by lifting a heavy weight a certain height. ( b ) In the quantum or micro-regime, we can think of work as the ability to excite a two-level system from one energy state to a higher one. Having many of these atoms would allow us to perform macroscopic work—for example, we could use the atoms in a laser. An amount of work W can be used to produce a transition from the state |00| to the state |11|, with Hamiltonian (we call such a two-level system the work qubit or wit). We can use such a system as a basic work storage unit, as our results will not depend on what physical system is used. Full size image Having precisely accounted for all sources of energy, we can apply techniques from single-shot information theory—a branch of information theory specializing in arbitrary resources as opposed to situations where we have many copies of independent and identically distributed bits of information (see, for example, Tomamichel [29] ). The techniques are thus ideally suited to the case where we want to extract work from a small single system or one whose subsystems are highly correlated. It is also applicable when we wish to extract a deterministic amount of work rather than just extract it statistically, as we can do here by considering systems in contact with a large heat bath that diminish the effect of statistical fluctuations of the system. Extractable work In this more general setting, we show in Supplementary Note 4 that the quantity that replaces the Helmholtz free energy for calculating the extractable work in the quantum regime is where with P E =| E ›‹ E | is the state ρ decohered in the energy eigenbasis (that is, off-diagonal terms are set to zero), h ( ω , g , E i ) is 1 if energy level | g , E i › is populated and 0 otherwise. β is the inverse temperature, and k is Boltzmann’s constant. For microscopic systems, one can generically extract very little work deterministically without allowing a tiny probability ε of failing to draw work [23] . In Supplementary Note 4 , we consider this situation and show that a β-smoothed version of F min , called , gives the optimal and achievable amount of work extractable from the resource. Its expression is found in Supplementary Note 4 ( Supplementary Equation (S59) ) and in the special case that the Hamiltonian is trivial, H =0, it corresponds to the expression of Dahlsten et al . [23] In terms of information-theoretic quantities, we can write where is the min-relative entropy [30] , [31] with Π ω , the projector onto the support of ω and τ is the Gibbs state with partition function Z . The min-relative entropy and single-shot free energy has been independently introduced as a lower bound for work extraction from classical states using a model of a series of independent interactions with a heat bath [32] . In the thermodynamical limit, D min ( ρ || τ ) becomes [21] the relative entropy , which is equal to F ( ρ )− F ( τ ) ( [19] ). Thus, while the maximum amount of work W that can be extracted when a macroscopic system is in contact with a heat bath is W ( ρ )= F ( ρ )− F ( τ ), more generally it is and only in the thermodynamical limit do we recover the traditional result. Although F min looks very different to the Helmholtz free energy, it can be compared with it easily in the situation where the given state ρ has energy fluctuations δ E , which are small compared with the average energy as is the case with macroscopic thermodynamical systems. We then consider a version ρ ε of the state ρ , with the tails of weight ε removed (this is more or less what happens when we smooth F min as discussed in Supplementary Note 4 ) and find by Taylor expanding F min ( ρ ε ) around the mean energy and taking the zeroeth order approximation that We can now compare this with the Helmholtz free energy. In the case where the system is block-diagonal in the energy eigenbasis, that is, we have that ρ = ω . Then, for extensive systems and the case of many particles n , the quantity ln rank( ω ε ) = ln rank( ρ ε )≈ S ( ρ ) with ε going to zero exponentially fast in n . (For example, for many non-interacting subsystems, such as an ideal gas, we may take the system to be composed of many systems in state ρ n . We then obtain the classical results [21] , and the smoothed min and max entropies approach the von-Neumann entropy [33] ; for extensive, isotropic systems, correlations do not play a role in thermodynamical quantities, and related results hold.) We then have that equation (5) approaches the Helmholtz free energy. In general however, ln rank ( ρ ε ) is larger than the entropy S ( ρ ), especially in the case where we just have a single system in the micro-regime, meaning that is smaller than the free energy. The finite size of the system means that less work can be extracted. There is a second reason why a limitation exists on the amount of extractable work. A quantum system ρ need not be in the form of equation (6) and in particular can have off-diagonal terms connecting different energy eigenstates. However, it is not ρ that enters into equation (3), but rather the state ρ decohered in the energy eigenbasis, namely ω . Thus, to zeroeth order, rather than the rank of ρ ε replacing the entropy, it is the rank of ρ ε dephased in the energy eigenbasis that replaces the entropy. This quantity is generally larger than the rank of ρ ε , which is why for systems with quantum coherences of energy there is a further limitation on how much work can be extracted. As an example, consider the pure quantum state It has entropy and rank equal to zero. However, when dephased in the energy eigenbasis to produce ω , it becomes the Gibbs state if the energy levels are non-degenerate, and has free energy − kT ln Z , no work can be extracted from it, despite it having zero entropy. However, as we approach the thermodynamic limit, the coherences matter less and less, and the free energy in the quantum case approaches the free energy for classical states [21] and, again, F min approaches the Helmholtz free energy. Work of formation The fact that at the quantum or nanoscale one can not extract the work as given by the free energy implies that there is an inherent irreversibility in thermodynamic transformations. This can also be seen as follows—the maximum amount of work that can be extracted from a system ρ in contact with a heat bath is given by F ε min ( ρ )− F ε min ( τ ). In the process, the system is transformed from state ρ to the Gibbs state τ . But if we wish to use work to perform the reverse process, namely transform Gibbs states into ρ using work, then we show in Supplementary Note 4 that the amount of work that is required is with in the case where ρ is diagonal in the energy eigenbasis. Here, the infimum is taken over states || ρ ε − ρ ||≤ ε with the optimal smoothing given in Supplementary Note 4 . In the case where the Hamiltonian is trivial H =0, equation (8) can be interpreted as an upper bound on the amount of work that can be extracted [23] , which coincides with the fact that in such a case, we interpret it as the amount of work that was put into creating the state to begin with. Such an interpretation can also be given to equation (8) in the case of full thermodynamics with energy. Again, to compare this quantity to the Helmholtz free energy, it is worth looking at the zeroth order approximation after expanding in powers of δ E /‹ E ›. We find where p max is the largest probability. To zeroeth order, we see that is related to the of the density matrix, the Helmholtz free energy to the entropy of the density matrix, and to ln (1/ p max ). When all probabilities of a density matrix are roughly equal, as is the case for many non-interacting particles ρ n , then these three quantities are equal as well. However, in general, , so that at the nanoscale we can generally extract less work from a resource than is required to create the resource, leading to a fundamental irreversibility in thermodynamical processes. In terms of information-theoretic quantities, , where is the max-relative entropy [30] . As we approach the thermodynamic limit , reversibility is restored [21] . More general thermodynamical transformations More generally, we would like to have criteria that tells us whether one state can be transformed into another under some thermodynamical process. As we have seen, because of finite size or quantum effects, the decreasing of the free energy is not a valid criteria that determines whether a thermodynamic transition can occur. For transitions between a system ρ and a system σ , both diagonal in the energy eigenbasis, we can derive necessary and sufficient criteria, which we call thermo-majorization. It is based on the majorization condition for state transformations, which is a necessary and sufficient condition for state transformations under permutation maps. Its construction is given in Supplementary Note 2 , and we state the result in Fig. 2 . An alternative derivation of our thermo-majorization condition can be obtained by adapting results of Ruch and Mead, studied in the context of decoherence and a particular master equation [34] , [35] , [36] and combining them with our proof that Thermal Operations are Gibbs preserving ones given in Supplementary Note 6 (this latter result in the special case of a heat bath composed of many independent systems was provided in Janzing et al . [37] ). The derivation we present in Supplementary Note 2 is more direct, and proves the conjecture that the ‘mixing distance’ decreases in thermodynamical systems—a problem that has been open since 1975 (ref. 35 ). We are also able to prove the converse. 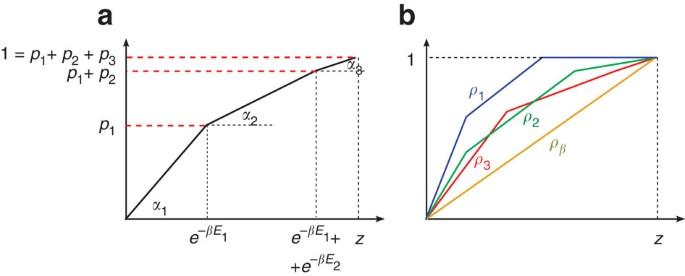Figure 2: Thermo-majorization. Consider probabilitiesp(E,g) of the initial systemρto be in theg'th state of energyE. Now let us putp(E,g)eβEin decreasing orderp(E1,g1)eβE1≥p(E2,g2)eβE2≥p(E3,g3)eβE3...—we say that the eigenvalues areβ-ordered. We can do the same for systemσ, that is,eβE1q(E1,g1) ≥eβE2q(E2,g2) ≥eβE3q(E3,g3).... Then the condition that determines whether we can transformρintoσis depicted in the above fig. Namely, (a) for any state, we construct a curve with pointskgiven by. Then (b) a thermodynamical transition fromρtoσis possible if and only if the curve ofρlies above the curve ofσ. One can make a previously impossible transition possible by adding work in the form of the pure stateψW, which will scale each point by an amounte−βWhorizontally. Figure 2: Thermo-majorization. Consider probabilities p ( E , g ) of the initial system ρ to be in the g 'th state of energy E . Now let us put p ( E , g )e βE in decreasing order p ( E 1 , g 1 ) e β E 1 ≥ p ( E 2 , g 2 ) e β E 2 ≥ p ( E 3 , g 3 ) e β E 3 ...—we say that the eigenvalues are β -ordered. We can do the same for system σ , that is, e β E 1 q ( E 1 , g 1 ) ≥ e β E 2 q ( E 2 , g 2 ) ≥ e β E 3 q ( E 3 , g 3 ).... Then the condition that determines whether we can transform ρ into σ is depicted in the above fig. Namely, ( a ) for any state, we construct a curve with points k given by . Then ( b ) a thermodynamical transition from ρ to σ is possible if and only if the curve of ρ lies above the curve of σ . One can make a previously impossible transition possible by adding work in the form of the pure state ψ W , which will scale each point by an amount e − βW horizontally. Full size image In the case where ρ is not diagonal in the energy eigenbasis, but the final state σ is diagonal, transformations are possible if and only if transformations are possible from ω to σ . The reason is simple—dephasing in the energy eigenbasis commutes with Thermal Operations [21] as the latter must conserve energy. As we can dephase the final state without changing it (as it is already diagonal in the energy basis), we can use the fact that dephasing commutes with our operations to instead dephase the initial state without changing whether the transformation is possible. In the case where the final state is also non-diagonal in the energy basis, the criteria for which transformations are possible depends on the coupling one has with the system and, especially, the degree of control one has of the system. Thus far, our results have not depended on having fine-grained control of the system and heat bath—the interaction depends on macroscopic variables such as total energy E , but the mapping between microstates g does not matter [21] . This is not necessarily the case during the formation process of states with off-diagonal terms. Thus, while equation (3) for the extractable work holds in general, the same is not true of equation (8) for the formation process. This is because for the formation process of transforming Gibb’s states into a state ρ that is not diagonal in the energy eigenbasis, it is generally not possible to make such a transformation using Thermal Operations without additional resources. In the case of formation of many copies n of ρ , the additional resource can be two-level pure states in a superposition of energy levels [21] , and the size of the system required scales sublinearly in n and hence vanishes as a fraction of n . In the case of a system of dimension two, we have derived necessary and sufficient conditions for a transformation to be possible, and necessary conditions in higher dimension. Changing Hamiltonians So far, we have considered transitions between the states of a system with fixed Hamiltonian. This might suggest that our approach does not cover the microscopic analogue of thermodynamical processes between equilibrium states with different initial and final Hamiltonians [3] , such as isothermal expansions of a gas in a container. Yet, fundamentally, a time-dependent Hamiltonian is only an effective picture of a fixed Hamiltonian of a larger system, and we shall show below how to describe such transitions in the microscopic regime. Namely, we introduce a qubit on system C that we can act on to switch the Hamiltonian from H to H ′ (we call this the switching qubit). We can, for example, take the total Hamiltonian to be and take the initial state of the work qubit, switching qubit and system to be |00›‹00| CW ρ and final state to be |11›‹11| CW σ , so that we are effectively changing the Hamiltonian acting on ρ , and gaining or losing work in the work qubit when we make the transition to σ . We now consider a transition between ρ and τ ′, the thermal state with Hamiltonian H ′, and want to know what value (positive or negative) for W allows us to make this transition. The results, obtained by means of thermo-majorization, are depicted in Fig. 3 . 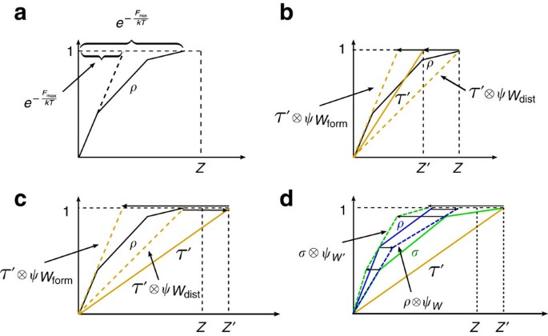Figure 3: Distillable work and work of formation. (a) Graphical representation of two free energies. For Gibbs state they coincide. (b,c) We can mimic the scenario of changing Hamiltonian by adding to the systemSancillaCswitching between initialHand final HamiltonianH′, with partition functionsZandZ′, respectively. We consider transitionρ→τ′ andτ′ →ρ, and obtainable works denote byWdistandWform, respectively. The works can be of either signs. Adding/subtracting work to a state is graphically represented as changing its slope. Formation is depicted by an arrow going fromρtoτ′, distillation by arrow going fromτ′ toρ. The directions of the arrow to the right/left means that the work is positive/negative in a given transition. Positive work means that we obtain work during the process. We depict two out of possible four cases of work signs: (b) both works are negative, (c) work of formation is negative while work of distillation is positive. (d) The interconversion of two arbitrary states is depicted by means of adding/subtracting work;Wis the maximal work that can be obtained by the transitionρ→σ;W′ is the minimal work needed to perform the transitionρ→σ. Hereis the excited state of the Hamiltonian, forE=W,W′,Wform,Wdist. One finds Figure 3: Distillable work and work of formation. ( a ) Graphical representation of two free energies. For Gibbs state they coincide. ( b , c ) We can mimic the scenario of changing Hamiltonian by adding to the system S ancilla C switching between initial H and final Hamiltonian H ′, with partition functions Z and Z ′, respectively. We consider transition ρ → τ ′ and τ ′ → ρ , and obtainable works denote by W dist and W form , respectively. The works can be of either signs. Adding/subtracting work to a state is graphically represented as changing its slope. Formation is depicted by an arrow going from ρ to τ ′, distillation by arrow going from τ ′ to ρ . The directions of the arrow to the right/left means that the work is positive/negative in a given transition. Positive work means that we obtain work during the process. We depict two out of possible four cases of work signs: ( b ) both works are negative, ( c ) work of formation is negative while work of distillation is positive. ( d ) The interconversion of two arbitrary states is depicted by means of adding/subtracting work; W is the maximal work that can be obtained by the transition ρ → σ ; W ′ is the minimal work needed to perform the transition ρ → σ . Here is the excited state of the Hamiltonian , for E = W , W ′, W form , W dist . Full size image for extracting work, and for the amount of work required to form ρ (provided it is diagonal in energy eigenbasis) from the thermal state, we obtain This result does not depend on the form of the Hamiltonian of equation (10)—we only require that at late times, there is no interaction between the work qubit and the other systems (as we need to be able to separate out the work qubit to use in some future process). More general state-to-state transformations assisted by work are also depicted. To derive equations (11) and (12), we β-order the p i and q i corresponding to ρ |00›‹00| and σ |11›‹11|, respectively. Then the thermo-majorization coordinates k of ρ |00›‹00| are given by , and those of σ |11›‹11| are . The thermo-majorization condition for a transition is that for all k , the points associated with ρ are above that of σ and they take a particularly simple form when either ρ or σ is the thermal state. These two cases are shown in Fig. 3 . The case where the final state is thermal for Hamiltonian H ′, σ = τ ′, and the work qubit is excited corresponds to distillation, as no further work can be drawn for fixed H ′ once the state is thermal, and a transition to another state can always be followed by a transition to the thermal state. Therefore drawing work by relaxing the state to a thermal state is completely general, and gives us equation (11). If ρ has off-diagonal terms, then the distillable work is given by the decohered version ω in equation (11), owing to the same reasoning as we used earlier—the final state is simply the work qubit, as everything else can be thrown away, and therefore is diagonal in the energy eigenbasis. As decohering the final state does not change the final state, and decohering with respect to the total Hamiltonian commutes with thermal operations, we can do it to the initial state without affecting the amount of work extractable. The case where we adjust W so that ρ |00›‹00| CW is thermo-majorized by σ |11›‹11| CW gives us the work required/distillable for a general transformation, while setting σ = τ gives the formation process and free energy of equation (12). The case where both initial and final states ρ and σ are thermal is also depicted in Fig. 3 , and leads to the ideal classical result, namely that a transition is possible if and only if that is, the work is given by the difference of standard free energies (1). Equation (13) is a very different result to equation (3), where we had no ancillary system isolated from the heat bath as in equation (10). It shows that for thermal equilibrium states there can be reversibility in some thermodynamical processes, provided they are between two thermal equilibrium states and the Hamiltonian changes. In the picture of a fixed Hamiltonian, this required at least one additional system (the switching qubit), which is effectively not in contact with the heat bath, and we do not draw the maximal amount of extractable work from the total working body, given by . The final state is thermal only on a subsystem S and therefore the amount of drawn work is not maximal. This strongly suggests that if we wish to carry out a Carnot cycle to extract work between two heat baths at different temperatures, then to get optimal efficiency during the isothermal process, we will need a working body of at least dimension 2 × 3. The first two-level system acts as the working body that interacts with the heat baths, while the additional three-level system is needed if we want to switch between different Hamiltonians in order to achieve the optimal isothermal work extraction given by equation (13). Even then, we find that while the two isothermal processes can be made ideal, the two adiabatic processes result in additional entropy production, meaning that the Carnot efficiency is not reached over a small number of cycles. This is analysed in Supplementary Note 7 . In general, we only get reversibility if there exists a W , such that the thermo-majorization plot of the initial state can get mapped onto the plot of the final state . Thus reversibility requires a very special condition. It is this lack of reversibility that requires two free energies. There is a connection here with other resource theories. Consider the set of states that are preserved under the class of operations—in entanglement theory, these are separable states, and for Thermal Operations, we show in Supplementary Note 6 that it is the Gibbs state. Now, if the theory is reversible, then under certain conditions, the relative entropy distance to the preserved set is the unique measure that governs state transformations [28] , [38] . For Thermal Operations, the relative entropy distance to the Gibbs state is precisely the free energy difference [19] . Here, in the case of finite sized systems, we see that although we do not have reversibility, the relative entropy distance to the preserved set again enters the picture, but it is the minimum and maximum relative entropy. These quantities are monotonically decreasing under the class of Thermal Operations, and provide two measures for state transitions. Proofs and derivations The proofs are contained in the Supplementary Information . In Supplementary Note 1 , we case thermodynamics as a resource theory, and in Supplementary Note 2 , we show that the condition for state transformations is given in terms of majorization. In Supplementary Note 3 , we consider transitions to and from pure states that we then use in Supplementary Note 4 to derive the extractable work and work of formation. Supplementary Note 5 discusses the case where we allow the use of ancillas and to what extent they can affect transition laws derived here. Supplementary Note 6 characterizes thermal operations, and looks at possible transitions in two- and three-level systems in the case where there are coherences between energy levels. Supplementary Note 7 discusses the details of a small engine undergoing a Carnot cycle. How to cite this article: Horodecki, M. & Oppenheim, J. Fundamental limitations for quantum and nanoscale thermodynamics. Nat. Commun. 4:2059 doi: 10.1038/ncomms3059 (2013).